Exciton dynamics reveal aggregates with intermolecular order at hidden interfaces in solution-cast organic semiconducting films Large-scale organic electronics manufacturing requires solution processing. For small-molecule organic semiconductors, solution processing results in crystalline domains with high charge mobility, but the interfaces between these domains impede charge transport, degrading device performance. Although understanding these interfaces is essential to improve device performance, their intermolecular and electronic structure is unknown: they are smaller than the diffraction limit, are hidden from surface probe techniques, and their nanoscale heterogeneity is not typically resolved using X-ray methods. Here we use transient absorption microscopy to isolate a unique signature of a hidden interface in a TIPS-pentacene thin film, exposing its exciton dynamics and intermolecular structure. Surprisingly, instead of finding an abrupt grain boundary, we reveal that the interface can be composed of nanoscale crystallites interleaved by a web of interfaces that compound decreases in charge mobility. Our novel approach provides critical missing information on interface morphology necessary to correlate solution-processing methods to optimal device performance. Small-molecule organic semiconductors are promising materials for thin film transistors, photovoltaics, displays and other printed electronics, but their complex film morphologies strongly impact their functionality [1] , [2] , [3] , [4] , [5] , [6] , [7] , [8] , [9] , [10] , [11] , [12] . In polycrystalline organic semiconducting thin films, grain boundaries are known to be strong inhibitors to charge transport as both a voltage barrier [2] , [12] , [13] , [14] , [15] , [16] and a possible location for trap states [12] , [14] , [15] , [16] , [17] , [18] . While it has been repeatedly shown that charge mobility is inversely proportional to the number of grain boundaries between electrical contacts [12] , [16] , [18] , [19] , there is still no consensus on the nature of the electronic structure of domain interfaces [20] , [21] , despite it being critical to device performance. Here we examine a domain interface in a drop-cast thin film of 6,13-bis(triisopropylsilylethynyl) pentacene (TIPS-Pn) (ref. 22 ), a material cited for high hole mobility [23] , [24] , [25] , [26] and singlet fission [27] , [28] , [29] , [30] . The crystal [31] and electronic [27] , [29] , [30] structure of the domains has been characterized, but analogous information for the domain interfaces is unknown. The difficulty in measuring the properties of these interfaces is twofold: surface probes such as atomic force microscopy cannot access an interface sandwiched between two domains, and the spatial resolution of traditional optical and X-ray diffraction techniques are insufficient to isolate interfacial signals. Nevertheless, we use a combination of transient absorption (TA) microscopy, with an optical focal volume ~1,000 times smaller than typical TA focal volumes, and a judicious selection of light polarization to isolate a signal at the interface that is not observed in either of the adjacent bulk domains. The exciton dynamics of this unique interfacial signal provide insight into its physical structure. TA microscopy has enabled the visualization of heterogeneity in the dynamic optical response within inorganic nanostructures [32] , [33] , [34] , [35] , [36] , polymer blends [37] and biological systems [38] , [39] . Previously, we used such an approach in thin films of TIPS-Pn (ref. 29 ), avoiding bulk averaging that can obscure the exciton dynamics occurring within individual crystalline domains. We found that the TA is highly sensitive to light polarization due to the anisotropy of the TIPS-Pn crystal structure. At the band edge, we observed a maximally negative excited-state absorption (ESA) TA signal when our probe light polarization was aligned with the long axis of the pentacenes. Conversely, we observed a maximally positive stimulated emission and/or ground state bleaching (GSB) TA signal when our probe light polarization was aligned with the short axis of the pentacenes (see Supplementary Note 1 ). We observed three dynamic processes, each on a distinct time scale, and proposed a model in which ultrafast relaxation of a hot excited singlet state occurred over tens of femtoseconds, an equilibrium between singlet fission and triplet annihilation occurred on a few-picosecond time scale, and internal conversion occurred over hundreds of picoseconds. This characterization of the exciton dynamics within individual crystalline domains provides a foundation for analyzing the TA signatures measured at their interface, which is the focus of this work. In what follows, we describe our observation of a TA signature that is specific to the interface between two large crystalline domains. By analyzing this signature, we determine that the region between these two domains has a finite, sub-diffraction extent. A structural model in which a collection of randomly oriented nanocrystallites are trapped in this region between domains is consistent with our observations. This kinetically trapped structure demonstrates an unintended consequence of solution processing that can begin to be addressed with the characterization that we provide. Studying the nature of domain interfaces constitutes a significant contribution towards achieving a complete picture of the correlation between structure and function in organic semiconducting films, and the approach that we demonstrate is applicable to a large variety of small-molecule materials being explored for high-mobility electronic applications. Unique TA signature observed at a domain interface The interrogated interface, in addition to portions of the two adjacent domains, underlies the TA measurement volume indicated with a red spot in Fig. 1a . TA measurements were also performed at the blue and green locations within each of the two adjacent bulk regions to aid in extracting the interfacial contribution to the TA measured in the red spot. Polarized linear absorption microscopy measurements [40] ( Supplementary Fig. 1 ) indicate that the interface is likely oriented diagonally relative to the substrate plane, as shown in the cross-section sketched in Fig. 1b . Analysis of high-numerical-aperture wide-field imaging of the film ( Supplementary Note 2 and Supplementary Fig. 2 ) indicates that the lateral extent of the interface is significantly smaller than the diffraction limit. If this interface were a molecularly abrupt grain boundary, it would consist of only ~1.8 × 10 6 interfacial molecules out of the ~1.8 × 10 9 included in the ~2 μm diameter TA interrogation volume of our 600-nm-thick film ( Supplementary Note 3 ). As such, by volume, a signal from the interface would represent only 0.1% of the total signal, while the remaining 99.9% would be attributed to the bulk crystalline domains adjacent to the boundary. Though we find that the interface is not molecularly abrupt, it is still remarkable that we are able to isolate the sub-diffraction interfacial contribution to the TA signal measured at the red spot. In addition to our spatial resolution, this isolation is possible because of the strong probe polarization dependence of the TA signal of each of the adjacent crystalline grains (blue and green traces in Fig. 2b ). 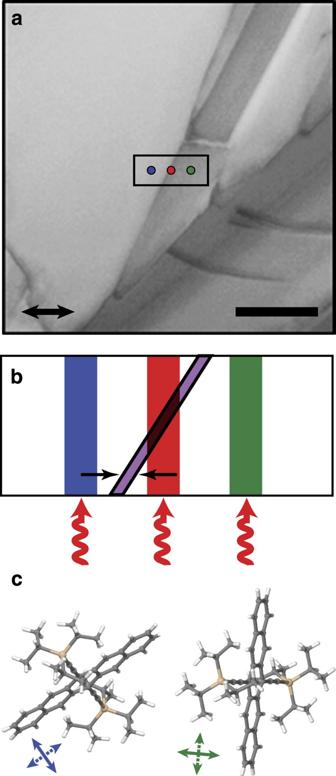Figure 1: Spatially resolved TA to uncover dynamics at a TIPS-Pn domain interface. (a) Wide field polarized transmission image of TIPS-Pn film with region-of-interest highlighted. Coloured spots mark the location of transient measurements. The double-headed arrow indicates 0° in the lab frame. Scale bar, 25 μm. (b) Schematic showing the interaction of the laser pulses with solely the left-hand domain, the interface and both domains and solely the right-hand domain at each of the measured spots. Arrows indicate the extent of the transverse cross-section of the interface (not to scale). (c) Orientation of the TIPS-Pn molecules in the crystalline domains represented in blue and green, projected into the substrate plane. Solid arrows indicate the orientation of the ground to S1transition dipole moment; dashed arrows indicate the orientation of the ESA transition dipole moment. Figure 1: Spatially resolved TA to uncover dynamics at a TIPS-Pn domain interface. ( a ) Wide field polarized transmission image of TIPS-Pn film with region-of-interest highlighted. Coloured spots mark the location of transient measurements. The double-headed arrow indicates 0° in the lab frame. Scale bar, 25 μm. ( b ) Schematic showing the interaction of the laser pulses with solely the left-hand domain, the interface and both domains and solely the right-hand domain at each of the measured spots. Arrows indicate the extent of the transverse cross-section of the interface (not to scale). ( c ) Orientation of the TIPS-Pn molecules in the crystalline domains represented in blue and green, projected into the substrate plane. Solid arrows indicate the orientation of the ground to S 1 transition dipole moment; dashed arrows indicate the orientation of the ESA transition dipole moment. 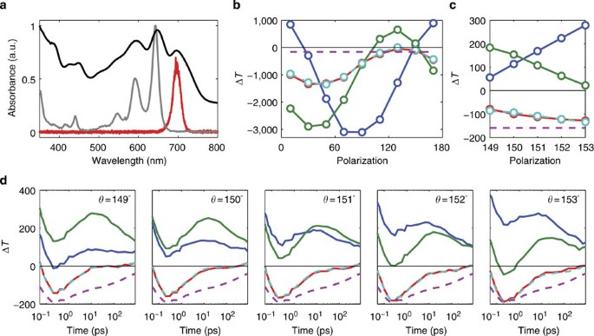Figure 2: TA signal of domain interface extracted using transients from adjacent grains. (a) Absorption spectrum of TIPS-Pn thin film (black) in toluene solution (grey) and the laser spectrum used for TA microscopy (red). (b) Dependence of TA signal at 1 ps on incident probe polarization with line colours corresponding to the spots inFig. 1a. Light blue dashed line isR′(θ,t) and purple line isI′(t). (c) TA signal as a function of probe polarization in the polarization range where bulk signal is near zero. (d) Transients measured at probe polarizations where bulk signal is near zero, and the calculatedR′(θ,t) andI′(t) transients at these polarizations. Full size image Figure 2: TA signal of domain interface extracted using transients from adjacent grains. ( a ) Absorption spectrum of TIPS-Pn thin film (black) in toluene solution (grey) and the laser spectrum used for TA microscopy (red). ( b ) Dependence of TA signal at 1 ps on incident probe polarization with line colours corresponding to the spots in Fig. 1a . Light blue dashed line is R ′( θ,t ) and purple line is I ′( t ). ( c ) TA signal as a function of probe polarization in the polarization range where bulk signal is near zero. ( d ) Transients measured at probe polarizations where bulk signal is near zero, and the calculated R ′( θ,t ) and I ′( t ) transients at these polarizations. Full size image At the locations indicated by the blue, green and red spots in Fig. 1a , TA at the TIPS-Pn 700-nm band edge was measured for probe polarizations from 10° to 170° in 20° steps in the lab frame, as shown in Fig. 3 . 0° in the lab frame is indicated by the double-headed arrow in Fig. 1a , and the molecular orientations in the crystalline domains on either side of the interface, projected in the sample plane, are shown in Fig. 1c , as determined by polarized linear absorption microscopy (see Supplementary Fig. 1 ). The transients measured in the homogeneously crystalline blue and green spots of Fig. 1a are similar to those presented in our previous work [29] . The time constants and amplitudes obtained from tri-exponential fits (~40 fs, 3 ps and 200 ps, with the amplitudes being positive, negative and decaying towards zero, respectively) indicate a similar crystal structure in the two domains adjacent to the interface. Fit parameters can be found in Supplementary Tables 1 and 2 . The transients in these two locations exhibit the periodic probe polarization dependences plotted in blue and green in Fig. 2b because of crystal anisotropy and a combination of orthogonal and competing resonant ground- and excited-state transition dipole moments both accessible to the probe pulse at 700 nm (see Supplementary Note 1 and ref. 29 ). The phase of this polarization dependence differs by ~50° between the two domains, owing to their crystal orientations being rotated relative to one another by ~50° in the substrate plane ( Fig. 1c ). As a result, the TA signal, Δ T , is minimized in both domains around a probe polarization of 150° ( Fig. 2c ). We have observed qualitatively similar behaviour in the TA of other interfaces and adjacent domains in films of TIPS-Pn; this coincident minimization of Δ T in both domains due to their relative orientation lies at the heart of our ability to identify an interface-specific TA signal. More generally, the occurrence of similar relative domain orientations throughout other polycrystalline small-molecule films is a common result of solution casting (see Supplementary Note 4 and Supplementary Fig. 3 ), and the minimization of Δ T that occurs when the ESA and GSB contributions overlap spectrally is a common phenomenon in the electronic structure of the polyacenes and their derivatives [27] , [29] , [41] , [42] , [43] , [44] , [45] and of other small molecules [46] , [47] , [48] being explored for high-mobility functions. We thus expect our interfacial characterization approach to be applicable to a broad class of relevant materials in present-day organic electronics, and this class will continue to expand, as developing new molecules [49] and extending domain sizes [26] , [50] are active areas of research. 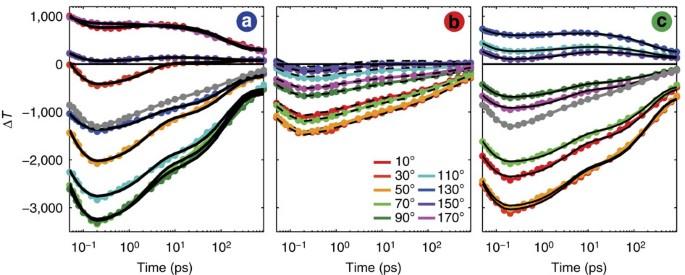Figure 3: Polarization-dependent transients and simultaneous fits. Coloured lines and data points are TA signal collected using different probe polarizations at the (a) blue spot, (b) red spot and (c) green spot inFig. 1a. Grey line is average of signal collected at all polarizations. Black lines inaandcare global fits of the data to a tri-exponential function. Dashed lines inbare fits of the data collected at the red spot to a weighted sum of the data collected at blue spot and the green spot, plus the extracted interfacial signal. Figure 3: Polarization-dependent transients and simultaneous fits. Coloured lines and data points are TA signal collected using different probe polarizations at the ( a ) blue spot, ( b ) red spot and ( c ) green spot in Fig. 1a . Grey line is average of signal collected at all polarizations. Black lines in a and c are global fits of the data to a tri-exponential function. Dashed lines in b are fits of the data collected at the red spot to a weighted sum of the data collected at blue spot and the green spot, plus the extracted interfacial signal. Full size image For most probe polarizations, the majority of the TA signal collected at the red spot in Fig. 1a originates from the molecules within the measurement volume that are part of the two large surrounding grains, shown schematically in Fig. 1b . By contrast, the existence of a unique interfacial signal is clearly observed in the set of transients presented in Fig. 2d , which were collected in 1° steps in the vicinity of 150°. In all of these plots, the signal collected from the location at the red spot is negative (dominated by ESA), while the signals collected within the adjacent grains are both positive (dominated by stimulated emission or GSB). Remarkably, it is impossible to construct the signal collected at the red spot that includes the interface by using a weighted sum of the blue and green signals collected wholly in each of the adjacent grains. Thus, the material at the interface must generate some negative contribution to the total signal that is different from the signals generated in the bulk of the adjacent grains. Isolating the TA contribution at a domain interface To consider the character of the interfacial exciton dynamics and its relation to morphology, the measured TA data at the red, blue and green spots were used to calculate I ′( t ), the TA signal generated by the molecules in the interfacial region only, which is plotted in purple in Fig. 2 . To do so, first, a weighted sum of the blue and green traces at each of the probe polarizations in Fig. 2d was subtracted from the corresponding red trace using a range of trial coefficient pairs between 0 and 1. For each pair of coefficients, the remaining, negative contribution to the red signal was identified as the potential interfacial contribution, I ′ trial ( t ). Second, for each set of trial coefficients, I ′ trial ( t ) and the corresponding weighted sum of the adjacent bulk domain contributions were used to reconstruct the entire, time-evolving TA signal at the red spot at all polarizations between 0–180° measured in Fig. 2b . This reconstruction, R ′( θ,t ), was compared with the measured signal R ( θ,t ), as shown in Supplementary Fig. 4 . The coefficients of the weighted sum that minimize the error of the reconstructed TA signal from the red spot simultaneously for all data collected between probe polarizations of 0 and 180° and at all time delays are 0.06±0.03 (blue) and 0.38±0.03 (green). Further details are presented in the Methods. Note, as elaborated in the Methods, that there are many more constraints than free parameters in this fitting procedure. Figure 3b and Supplementary Fig. 5 show R ( θ,t ), the measured TA signals at the red spot for these probe polarizations (coloured) and the excellent simultaneous agreement of R ′( θ,t ), the corresponding reconstructed transients (black) when these optimal coefficients are used. Deviating from the optimal coefficients introduces far poorer agreement, as illustrated in Supplementary Fig. 6 . The time constants of tri-exponential fits to I ′( t ), <B ( t ) > and <G ( t ) > are presented in Table 1 , where <B ( t ) > and <G ( t ) > represent transients averaged over all collected probe polarizations in each of the adjacent domains (grey lines in Fig. 3 ), and shed light on the nature of the interface between grains. Notably, the transients at the interface (purple in Fig. 2d ) have nearly identical time constants to those observed in the bulk crystalline domains (blue and green). This suggests that the corresponding detected excited-state processes, which are highly sensitive to molecular configuration [25] , [26] , [51] , [52] , are likely the same at the interface and in the bulk regions. This indicates that the TIPS-Pn molecules that contribute to the extracted interfacial signal exist in a local environment similar to those in the surrounding bulk crystalline regions. To support bulk exciton dynamics, the local intermolecular order in the interfacial region must extend over distances at least greater than several molecules’ extent, implying also that the interfacial region has a finite width. Table 1 Fit time constants of I ′( t ), <B ( t ) > and <G ( t ) > . Full size table As further support of this crystallinity, note that we pump and probe at the 700 nm band edge of crystalline TIPS-Pn, whereas the lowest energy absorption peak in amorphous TIPS-Pn thin films is at 645 nm (ref. 53 ), which is not resonant with our laser excitation ( Fig. 2a ). The red-shift of the band edge in the polycrystalline film indicates that the solid state exciton is stabilized by the surrounding TIPS-Pn molecules in an ordered film and is likely delocalized. Thus, the detection of TA from the interfacial region using a 700 nm excitation and probe is further evidence that the molecules in this region maintain a similar crystal structure to those in the bulk. Since the correlation length of intermolecular order is too small to be resolved by traditional characterization techniques, we consider the possible models that are consistent with our data. There are three qualitatively different categories of possible interface morphology, each illustrated in Fig. 4 , that could be consistent with the above evidence of crystallinity. If the interface were composed of a single, narrow crystalline domain ( Fig. 4b , purple), the interfacial signal would have a significant polarization dependence, requiring additional parameters in our fitting process. Since we can successfully extract I ′( t ) without introducing these additional parameters, it is more likely that many possible molecular orientations are present in the interfacial region. The two extremes of intermolecular order that support multiple molecular orientations are shown in Fig. 4a,c . In Fig. 4c , the molecular orientation varies slowly yet continuously to bridge the region between the two larger crystalline domains in blue and green. The electrostatic interaction between neighbouring molecules in this particular configuration would not be as favourable as in a proper crystal lattice. This state is both entropically and enthalpically disfavoured and is unlikely to be kinetically trapped during solution casting. This motif would thus extend only over very short distances [54] , [55] , such that the interfacial contribution to the TA would become much smaller than we measure (see discussion below about the size of I ′). It is therefore more likely that there are multiple nanoscale crystalline domains with different orientations present in the interfacial region. 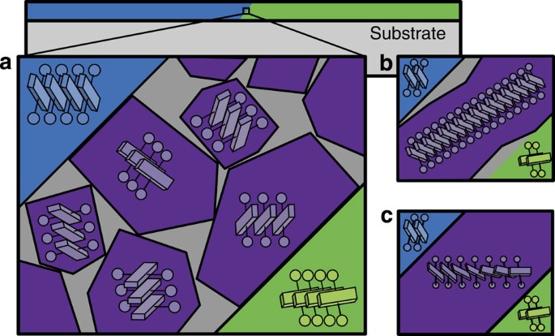Figure 4: Model of structure at domain interface. (a) Sketch of a structure in which the interfacial region between the larger domains (represented in blue and green) consists of small, nano-crystalline domains (purple) consistent with the measured TA data. The grey interstices do not generate a TA signal at 700 nm and could be voids or amorphous regions. This structure is hidden beneath the surface of the film and is not accessible to surface probes. Alternative, though less likely, structures could involve (b) a single crystalline domain at the interface, or (c) an interstitial region in which the molecular orientation varies smoothly. Figure 4: Model of structure at domain interface. ( a ) Sketch of a structure in which the interfacial region between the larger domains (represented in blue and green) consists of small, nano-crystalline domains (purple) consistent with the measured TA data. The grey interstices do not generate a TA signal at 700 nm and could be voids or amorphous regions. This structure is hidden beneath the surface of the film and is not accessible to surface probes. Alternative, though less likely, structures could involve ( b ) a single crystalline domain at the interface, or ( c ) an interstitial region in which the molecular orientation varies smoothly. Full size image A cartoon of this more likely physical structure consistent with our observations is highlighted in Fig. 4a . We depict the cross-section of the interfacial region with a mixture of isotropically oriented nanoscale crystalline regions (purple) surrounded by more disordered regions and/or voids (grey). Such a structure could develop during solution casting from the accumulation of small aggregates between the larger (blue and green) domain crystallization fronts as the solvent evaporates [56] . The presence of regions of additional disorder between these nanoscale grains would be a response to the presence of high energy interfaces and kinetic trapping of molecules away from equilibrium positions [54] , [55] , [57] , [58] , [59] . Since I ′( t ) exhibits the same dynamics as the TA signal at the bulk locations, we attribute the unique TA signal that we have observed at the interface to the trapped purple nanoscale grains and not to any intervening disordered regions or molecularly abrupt grain boundaries. The idea that interfaces between grains in TIPS-Pn may have a finite width as previously suggested by Wo et al . [12] , who concluded that these boundaries must have a width of at least 10 nm to sustain the electric field associated with a measured voltage drop between grains without inducing molecular breakdown. Here we consider the relative strength of the I ′( t ) signal compared with the bulk domain signals to estimate the spatial extent of our measured interfacial region. The extracted interfacial TA signal I ′( t ) in Fig. 2d is on average ~15% of the magnitude of the polarization-averaged signal strengths <B ( t ) > and <G ( t ) > from the two adjacent grains in Fig. 3a,c . This is much larger than would be expected if the interface between the two grains were a molecularly abrupt boundary. Crystallites templated on the glass substrate generally maintain an angle of 26° between the S 0 −S 1 transition dipole moment and the normal to the substrate plane [31] . By contrast, for a collection of isotropically oriented nanocrystals, we compute that the pump excitation field will couple 56% more strongly to the S 0 −S 1 transition dipole moments. Accounting for this orientation factor, our findings suggest that the interface region could be laterally at most ~200 molecules wide (see Supplementary Note 5 ). Based on an average molecular spacing of 7.8 Å in the a–b plane [22] , [31] , this corresponds to a sub-diffraction width of ~150 nm. Thus, by spectrally selecting for aggregates which can sustain bulk excitons, our spatially resolved TA measurements have enabled us to infer sub-diffraction structural properties at a hidden interface between domains. This interface cannot be accessed using surface techniques such as atomic force microscopy or microbeam grazing incidence wide-angle X-ray scattering [60] and would be extremely challenging to characterize using scanning transmission X-ray microscopy, which integrates over the thickness of the film [61] , [62] , [63] . In sum, our measurements show that the interfacial region between crystal grains in solution-cast films of TIPS-Pn can have a finite extent in which the molecules maintain a crystal packing similar to that in the large adjacent bulk regions, yet over length scales that are smaller than the diffraction limit. The spectral and temporal properties of the TA signature that we isolate at this type of interface suggest that it is composed of nanocrystallites that may have become kinetically trapped during solution casting between two crystallization fronts. Our findings indicate that solution-cast films may contain far more grain boundaries than anticipated when an interfacial region is composed of a random packing of nanocrystallites. These discontinuities can strongly affect the transport properties of films in device applications. Our unique ability to uncover structural motifs at a hidden interface will therefore significantly advance the ability to systematically determine the optimal casting conditions to control intricate morphology and resulting functional properties in organic electronics. For example, our measurements should lend predictive power to scalable and affordable solution-processing approaches to minimize discontinuities and maximize charge mobility. Further extending these measurements to excite sub-diffraction optical volumes would enable studies of film morphologies with higher degrees of disorder, as is the case in polymeric materials and their heterojunctions. Film preparation and characterization As in ref. 29 , filtered (0.2 μm pore size) 5 mg per ml solutions of TIPS-Pn in toluene were dropcast onto clean glass substrates on top of a hotplate held at ~60 °C. After deposition, samples were covered with a Petri dish to control solvent evaporation rate. For this study, film deposition was conducted in a glove box using dry toluene. This yielded ~600-nm-thick films with finger-like domains 10–150 μm wide and up to hundreds of microns long. Samples were removed from the glove box and mounted face down onto large rectangular coverslips. TA microscopy TA microscopy measurements were conducted in a home-built optical microscope [29] . Briefly, 5 kHz, 700 nm center-wavelength laser pulses were used to pump the S 0 →S 1 transition of TIPS-Pn ( Fig. 3a ). The beam was split into degenerate pump and probe pulses in a 4:1 intensity ratio and focused on the sample using a 0.4 NA objective to yield full-width half-maximum (FWHM) spot sizes of ~4 μm and pulse durations of ~35 fs. This results in an optical volume which is ~1,000 times smaller than in a typical bulk TA experiment where a 100–200 μm FWHM spot is used. Since TA is a non-linear process requiring three light-matter interactions, the effective measurement volume diameter is ~2 μm (FWHM). Energy fluences of 400 μJ cm −2 and 100 μJ cm −2 for the pump and probe were used, which avoids photodamage and exciton annihilation (see Supplementary Note 6 ). Probe polarizations were varied by rotating a motorized waveplate. After passing through the sample, the transmitted beams were collected using a second, identical objective and the pump beam was removed via spatial filtering. The probe signal was focused onto a photomultiplier tube. The output from the photomultiplier tube was coupled to a lock-in amplifier, locked to the pump chopping frequency (500 Hz), to collect the unnormalized TA signal, Δ T. Typically, Δ T is divided by the linear transmission T to obtain the differential optical density, independent of incident light intensity. In this study, however, we analyze Δ T alone because this differential measurement eliminates time-independent scatter from the strongly scattering interface, while T does not. To analyze Δ T/T would convolve absorption and scatter over the entire measurement volume that contains the interface and surrounding domains. By rastering the sample position using a computer controlled Physik Instrumente piezostage, Δ T was collected at multiple spatial locations. For each time delay, polarization and spatial location, the reported signal is the average of 18,750 pulses. Polarized linear absorption microscopy By toggling kinematically mounted mirrors, the optical microscope could be modified to use a white light emitting diode (Thorlabs MWWHL3) as an illumination source. The light passed through a 700 nm bandpass filter (Thorlabs FB700-10) and a polarizer before reaching the sample, and the transmitted light was imaged onto a CMOS camera (Thorlabs DCC1545M). Wide field transmission images of the sample were collected in 5° polarization increments. Extraction of interface TA signal In the following, variables with a prime indicate calculated values, while those without a prime denote measured TA data. The data collected near probe polarization θ =150° are used to extract the signal specific to the interface using for θ =149°–153° where I ′ is the signal generated in the interfacial region, and R , B and G are the signals measured at the red, blue and green spots in Fig. 1a , respectively. The coefficients c 1 and c 2 define the weighted sum of the contribution to the signal in the red spot that comes from the two adjacent grains. I ′ trial was calculated for all possible combinations of c 1 and c 2 from 0 to 1 (that is, from no to full relative contribution) in steps of 0.001. For each combination of c 1 and c 2 , the I ′ trial ( t ) transient functions calculated at each polarization from 149° to 153° ( Supplementary Fig. 7 ) were averaged together to yield <I ′ > ( t ), shown in dashed purple in Fig. 2d , and this averaged function was used to calculate a reconstruction, R ′, of the TA signal measured at the red spot for the full range of all measured probe polarizations θ =0°–180°, R ′ is plotted in dashed cyan in Fig. 2 . Here R ′ uses the weighted sum defined by c 1 and c 2. The difference between the reconstructed signal R ′ and the measured signal R was determined for every combination of c 1 and c 2 . The coefficients that yielded the minimum absolute difference between R and R ′, integrated over all measured probe polarization angles and time delays, were determined to be c 1 =0.061 and c 2 =0.383. The above procedure involves finding the best fit of a function I ′( t ) and two constant coefficients, c 1 and c 2 to our data set according to equations 1 and 2. While this involves a total set of free parameters equal to the number of time points plus the two coefficients, the effective number of constraints applied is equivalent to the total number of independent equations of the form of equation 2 for each pair of the variables θ and t . In other words, since we use information from a total of nine different probe polarizations, there are nine times as many constraints as free parameters in the fitting procedure. How to cite this article: Wong, C. Y. et al . Exciton dynamics reveal aggregates with intermolecular order at hidden interfaces in solution-cast organic semiconducting films. Nat. Commun. 6:5946 doi: 10.1038/ncomms6946 (2015).